Orai1-dependent calcium entry promotes skeletal muscle growth and limits fatigue Store-operated Ca 2+ entry (SOCE) in skeletal muscle involves signalling between stromal-interacting molecule 1 (STIM1) in the sarcoplasmic reticulum (SR) and Ca 2+ selective Orai1 channels in the sarcolemma. Here we generate transgenic mice with muscle-specific expression of dominant-negative Orai1 (dnOrai1) and demonstrate that Orai1-dependent SOCE promotes growth and limits fatigue in adult skeletal muscle. dnOrai1 mice lack SOCE specifically in muscle but are fertile and thrive well into adulthood. Although muscle ultrastructure, excitation–contraction (EC) coupling, fibre type, and expression of other Ca 2+ regulatory proteins are unaltered, dnOrai1 mice exhibit reduced body weight, muscle mass and fibre cross-sectional area. Importantly, during intense repetitive activity, dnOrai1 mice display increased susceptibility to fatigue at the single fibre, excised muscle and whole-animal levels. We further show that STIM1 and Orai1 proteins co-localize within the triad junction but do not exist in a preassembled context. These results show that Orai1-dependent SOCE has an important physiological role in muscles of adult mice. Store-operated Ca 2+ entry (SOCE) is activated by depletion of intracellular Ca 2+ stores [1] . In non-excitable cells, SOCE is coordinated by stromal-interacting molecule 1 (STIM1) serving as an endoplasmic reticulum (ER) Ca 2+ sensor [2] , [3] , [4] that activates Ca 2+ -selective Orai1 channels in the plasma membrane [5] , [6] . Specifically, store depletion results in Ca 2+ unbinding from the luminal EF hand (helix-loop-helix) motif of STIM1, which induces STIM1 aggregation and translocation to adjacent ER plasma membrane junctions. Within these junctions, STIM1 aggregates interact with Orai1 to activate the channel and promote Ca 2+ influx [7] , [8] , [9] , [10] . SOCE in skeletal myotubes exhibits a similar biophysical, pharmacological and molecular signature as that observed in non-excitable cells. SOCE in myotubes is activated by depletion of SR Ca 2+ stores and is inhibited by multiple SOCE inhibitors including lanthanide, BTP-2, 2-APB and SK&F-96365 (refs 11 , 12 , 13 , 14 ). SOCE in myotubes depends on STIM1–Orai1 coupling as it is abolished by both STIM1 knockdown and expression of human dominant-negative Orai1 (dnOrai1; E106Q) [12] , [14] , [15] . SOCE is also absent in myotubes derived from mice with global [13] or skeletal muscle-specific [11] deletion of STIM1. Finally, voltage clamp studies [14] indicate that the SOCE channel current in myotubes exhibits similar biophysical, pharmacological and molecular properties as that observed in T lymphocytes [16] , [17] . Although SOCE in muscle has been linked to Ca 2+ store repletion [18] , fatigue [19] , [20] , NFAT transactivation [13] , [21] and muscle differentiation [11] , [13] , [22] , the precise physiological role(s) of STIM1–Orai1 coupling and Orai1-dependent Ca 2+ entry in adult skeletal muscle remains unclear. Rosenberg et al . [21] reported that global and muscle-specific STIM1 ablation results in a profound reduction in muscle mass, a severe myopathy and neonatal lethality [11] , [13] . However, STIM1 is a multipurpose stress transducer activated by diverse stimuli (depletion, oxidation, temperature, hypoxia and acidification) that regulates multiple targets including channels (Orai1, TrpC, ARC and Cav1.2), pumps/exchangers (Sarco-Endoplasmic Ca 2+ ATPase (SERCA), Plasma membrane Ca 2+ ATPase (PMCA), Na/Ca exchanger), adaptor proteins (POST), ER chaperones (calnexin and ERp57), signalling enzymes (adenylate cyclase isoform 8) and ER stress/remodelling proteins (microtubule protein EB1) [23] . Thus, the specific role of STIM1–Orai1 coupling in the survival and complex muscle phenotypes of STIM1 knockout mice is unclear. To determine the role of Orai1-dependent Ca 2+ entry in skeletal muscle structure and function, we generated transgenic mice with muscle-specific expression of dnOrai1 mice. Remarkably, unlike STIM1 knockout mice, dnOrai1 mice are viable, fertile and live a normal lifespan. Thus, dnOrai1 transgenic mice enabled determination of the specific role of Orai1-dependent Ca 2+ entry in skeletal muscle growth, development and performance in adult animals. STIM1 and Orai1 do not form preassembled triad complexes Although STIM1–Orai1 coupling underlies SOCE in myotubes, this has not been rigorously determined in fully differentiated adult skeletal muscle fibres. Using immunocytochemical studies in single mouse flexor digitorum brevis (FDB) fibres from adult mice, Orai1 exhibited a double-row pattern of fluorescence that co-localized with the ryanodine receptor ( Fig. 1a ), confirming the presence of Orai1 within the triad junction. STIM1 fluorescence was observed throughout the I-band region, flanking discrete Z-disk localization α-actinin, although also significantly enriched with RyR1 in the triad ( Fig. 1b,c ). Co-localization of STIM1 and Orai1 in the triad of resting muscle fibres is consistent with a uniquely extremely rapid (for example, tens of milliseconds) and efficient SOCE activation on SR Ca 2+ store depletion in muscle [14] , [24] , [25] , [26] . To support such rapid activation, STIM1 and Orai1 have been proposed to be closely associated or even form preassembled complexes that are directly activated on store depletion [25] , [27] . This hypothesis was tested using bimolecular fluorescence complementation (BiFC) [28] , [29] , [30] to determine whether junctional STIM1 and Orai1 proteins form preassembled SOCE channel complexes in fibres with fully replete SR Ca 2+ stores. FDB muscles were electroporated with complementary DNAs encoding cherry-STIM1-N (1–158) YFP and cherry-Orai1-C (159–283) YFP. Although expressing fibres lacked basal yellow fluorescent protein (YFP) fluorescence, robust junctional YFP fluorescence was observed following thapsigargin (TG)-induced store depletion ( Fig. 1d,e ). Thus, although STIM1 and Orai1 co-localize in the triad, they do not form preassembled STIM1–Orai1 complexes in the absence of SR store depletion. 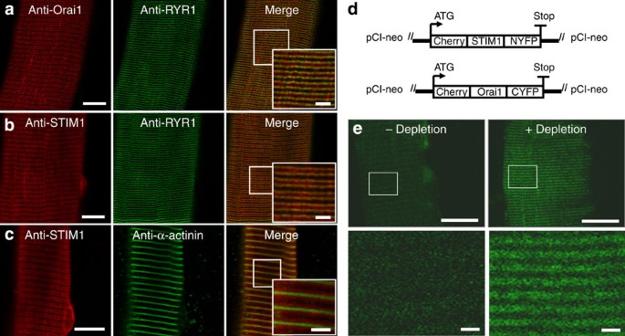Figure 1: Co-localization of endogenous STIM1 and Orai1 at the triad junction and formation of STIM1–Orai1 complexes on store depletion. (a) Representative immunofluorescence images of endogenous Orai1 alone (left), RyR1 alone (middle) and overlay (right) in a FDB fibre from an adult WT mouse. (b) Representative immunofluorescence images of endogenous STIM1 alone (left), RyR1 alone (middle), and overlay (right) in a FDB fibre from an adult WT mouse. (c) Representative immunofluorescence images of endogenous STIM1 alone (left), α-actinin alone (middle) and overlay (right) in a FDB fibre from an adult WT mouse. Scale bars, 10 μm for low-magnification images and 2 μm for high-magnification images. (d) Schematic maps of split YFP constructs used in BiFC experiments. The amino-terminal fragment of YFP (1–158) was fused to the C terminus of cherry-tagged STIM1 (top) and the C-terminal YFP fragment (159–238) was fused to the C terminus of cherry-tagged Orai1 (bottom). (e) Top: representative images of YFP fluorescence in FDB fibres expressing cherry-STIM1-NYFP and cherry-Orai1-CYFP before (left) after (right) TG-induced store depletion. Scale bars, 10 μm. (Bottom) Higher-magnification images in the boxed regions shown in the top panels. Scale bars, 2 μm. Figure 1: Co-localization of endogenous STIM1 and Orai1 at the triad junction and formation of STIM1–Orai1 complexes on store depletion. ( a ) Representative immunofluorescence images of endogenous Orai1 alone (left), RyR1 alone (middle) and overlay (right) in a FDB fibre from an adult WT mouse. ( b ) Representative immunofluorescence images of endogenous STIM1 alone (left), RyR1 alone (middle), and overlay (right) in a FDB fibre from an adult WT mouse. ( c ) Representative immunofluorescence images of endogenous STIM1 alone (left), α-actinin alone (middle) and overlay (right) in a FDB fibre from an adult WT mouse. Scale bars, 10 μm for low-magnification images and 2 μm for high-magnification images. ( d ) Schematic maps of split YFP constructs used in BiFC experiments. The amino-terminal fragment of YFP (1–158) was fused to the C terminus of cherry-tagged STIM1 (top) and the C-terminal YFP fragment (159–238) was fused to the C terminus of cherry-tagged Orai1 (bottom). ( e ) Top: representative images of YFP fluorescence in FDB fibres expressing cherry-STIM1-NYFP and cherry-Orai1-CYFP before (left) after (right) TG-induced store depletion. Scale bars, 10 μm. (Bottom) Higher-magnification images in the boxed regions shown in the top panels. Scale bars, 2 μm. Full size image Characterization of SOCE in adult skeletal muscle fibres We used Mn 2+ quench of fura-2 fluorescence [12] to examine the molecular determinants and pharmacological signature of SOCE in FDB fibres from adult mice. Although fura-2 emission was unaltered during application of extracellular Mn 2+ in non-depleted fibres ( Fig. 2a ), a significant increase in fura-2 quench rate was observed in TG-treated fibres ( Fig. 2b ), consistent with robust SOCE activation. Mn 2+ quench in store-depleted fibres was inhibited by addition of either 0.2 mM LaCl 3 or 10 μM BTP-2 ( Fig. 2c,d ). To assess the importance of Orai1 in this store-dependent entry, cherry-tagged mouse dnOrai1E108Q was transiently expressed by electroporation in FDB muscles of adult mice. TG-pretreated, E108Q-expressing fibres lacked a significant change in fura-2 quench on addition of extracellular Mn 2+ ( Fig. 2e ). Electroporation of FDB muscles with a mixture of four STIM1-specific short-interfering RNAs (siRNAs), but not negative control siRNAs ( Supplementary Table S1 ), markedly reduced expression of both short (average±s.e.m. : 62±12%) and long (average±s.e.m. : 80±5%) STIM1 isoforms ( Supplementary Fig. S1 ). STIM1 knockdown abolished Mn 2+ quench in FDB fibres following store depletion ( Fig. 2f ), whereas no effect was observed for negative control siRNAs ( Fig. 2g ). Average (±s.e.m.) values for the maximal rate of Mn 2+ quench for the conditions shown in Fig. 1a–g are summarized in Fig. 1h . These results demonstrate that SOCE in adult skeletal muscle requires STIM1–Orai1 coupling and that this process is abolished by the expression of dnOrai1. 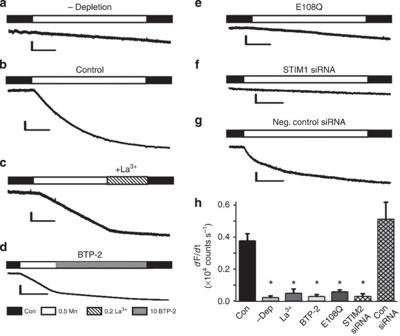Figure 2: SOCE in adult skeletal muscle depends on STIM1–Orai1 coupling. (a) Representative Mn2+quench trace in an adult FDB fibre in the absence of store depletion. (b–g) Representative Mn2+quench traces in adult FDB fibres obtained following TG-induced store depletion in control (b), during addition of 200 μM La3+(c), during addition of 10 μM BTP-2 (d), following expression of cherry-tagged E108Q (e), STIM1 siRNAs (f) or negative control siRNAs (g). (h) Average (±s.e.m.) maximum rate of Mn2+quench in the absence of store depletion (−Dep,n=4) and following TG-induced store depletion in control (Con,n=29), 200 μM La3+(n=4), 10 μM BTP-2 (n=10), cherry-tagged E108Q expression (n=12), STIM1 siRNAs (n=8) and negative control siRNAs (n=9). *P<0.01 compared with control by analysis of variance andpost hocStudent–Newman–Keuls test. Scale bars, 100 s (a–e), 50 s (f,g) (horizontal); 0.2 × 106counts (a–e), 0.1 × 106counts (f,g) (vertical). Figure 2: SOCE in adult skeletal muscle depends on STIM1–Orai1 coupling. ( a ) Representative Mn 2+ quench trace in an adult FDB fibre in the absence of store depletion. ( b – g ) Representative Mn 2+ quench traces in adult FDB fibres obtained following TG-induced store depletion in control ( b ), during addition of 200 μM La 3+ ( c ), during addition of 10 μM BTP-2 ( d ), following expression of cherry-tagged E108Q ( e ), STIM1 siRNAs ( f ) or negative control siRNAs ( g ). ( h ) Average (±s.e.m.) maximum rate of Mn 2+ quench in the absence of store depletion (−Dep, n =4) and following TG-induced store depletion in control (Con, n =29), 200 μM La 3+ ( n =4), 10 μM BTP-2 ( n =10), cherry-tagged E108Q expression ( n =12), STIM1 siRNAs ( n =8) and negative control siRNAs ( n =9). * P <0.01 compared with control by analysis of variance and post hoc Student–Newman–Keuls test. Scale bars, 100 s ( a – e ), 50 s ( f , g ) (horizontal); 0.2 × 10 6 counts ( a – e ), 0.1 × 10 6 counts ( f , g ) (vertical). Full size image Effect of SOCE on Ca 2+ transients during tetanic stimulation As SR Ca 2+ stores in FDB fibres are significantly reduced during a single high-frequency stimulation train [31] , we determined the effect of inhibiting SOCE on myoplasmic Ca 2+ transients elicited by multiple repetitive, high-frequency tetanic stimulation trains ( Fig. 3 ). Myoplasmic Ca 2+ transients were monitored in single FDB fibres using mag-fluo-4, a rapid, low-affinity Ca 2+ dye that maximizes resolution of Ca 2+ transient magnitude and kinetics [32] . Mag-fluo-4-loaded fibres were stimulated for 60 consecutive tetanic trains (500 ms, every 2.5 s, at 50 Hz, 60 times). Ca 2+ transient magnitude during each tetani and the integral of the decaying phase of the Ca 2+ transient (‘tail Ca 2+ transient integral’) following termination of each train were quantified ( Supplementary Fig. S2a ). 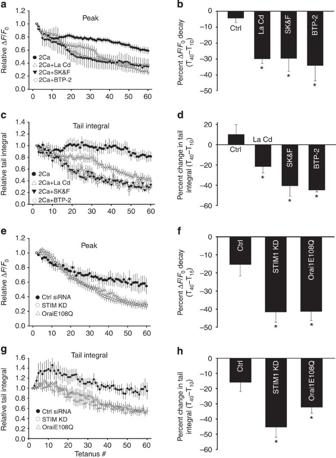Figure 3: SOCE maintains Ca2+transient amplitude during repetitive tetanic stimulation. (a) Average (±s.e.m.) peak Ca2+transient amplitude during 60 consecutive tetanic stimuli (500 ms, at 50 Hz, every 2.5 s) in control (2 Ca2+, filled circles,n=14) or in the presence of 200 μM La3+plus 500 μM Cd2+(open triangles,n=15), 30 μM SK&F-96365 (inverted-filled triangles,n=5) or 10 μM BTP-2 (open circles,n=6). (b) Average (±s.e.m.) percent reduction in peak Ca2+transient amplitude from tetanus 10 to tetanus 40 ([T40−T10] × 100) in the absence and presence of blockers. (c) Average (±s.e.m.) relative Ca2+transient tail integral after each tetani for the experiments in shown ina. (d) Average (±s.e.m.) percent change in Ca2+transient tail integral ([T40−T10] × 100) for the experiments shown inc. (e) Average (±s.e.m.) peak Ca2+transient amplitude during 60 consecutive tetanic stimuli (500 ms at 50 Hz every 2.5 s) in FDB fibres treated with either negative control siRNA (Ctrl siRNA, filled circles,n=10), STIM1-targeted siRNA (STIM KD, open circles,n=18) or expressing cherry-tagged Orai1E108Q cDNA (open triangles,n=5). (f) Average (±s.e.m.) percent reduction in peak Ca2+transient amplitude from tetanus 15 to tetanus 40 ([T40−T15] × 100) in FDB fibres treated with negative control siRNA or STIM1-targeted siRNA or Orai1E108Q cDNA. (g) Average (±s.e.m.) relative Ca2+transient tail integral for the experiments shown ine. (h) Average (±s.e.m.) percent reduction in Ca2+transient tail integral ([T40−T10] × 100) for the experiments shown ing. *P<0.05 compared with control by analysis of variance andpost hocStudent–Newman–Keuls test. Figure 3: SOCE maintains Ca 2+ transient amplitude during repetitive tetanic stimulation. ( a ) Average (±s.e.m.) peak Ca 2+ transient amplitude during 60 consecutive tetanic stimuli (500 ms, at 50 Hz, every 2.5 s) in control (2 Ca 2+ , filled circles, n =14) or in the presence of 200 μM La 3+ plus 500 μM Cd 2+ (open triangles, n =15), 30 μM SK&F-96365 (inverted-filled triangles, n =5) or 10 μM BTP-2 (open circles, n =6). ( b ) Average (±s.e.m.) percent reduction in peak Ca 2+ transient amplitude from tetanus 10 to tetanus 40 ([T 40 −T 10 ] × 100) in the absence and presence of blockers. ( c ) Average (±s.e.m.) relative Ca 2+ transient tail integral after each tetani for the experiments in shown in a . ( d ) Average (±s.e.m.) percent change in Ca 2+ transient tail integral ([T 40 −T 10 ] × 100) for the experiments shown in c . ( e ) Average (±s.e.m.) peak Ca 2+ transient amplitude during 60 consecutive tetanic stimuli (500 ms at 50 Hz every 2.5 s) in FDB fibres treated with either negative control siRNA (Ctrl siRNA, filled circles, n =10), STIM1-targeted siRNA (STIM KD, open circles, n =18) or expressing cherry-tagged Orai1E108Q cDNA (open triangles, n =5). ( f ) Average (±s.e.m.) percent reduction in peak Ca 2+ transient amplitude from tetanus 15 to tetanus 40 ([T 40 −T 15 ] × 100) in FDB fibres treated with negative control siRNA or STIM1-targeted siRNA or Orai1E108Q cDNA. ( g ) Average (±s.e.m.) relative Ca 2+ transient tail integral for the experiments shown in e . ( h ) Average (±s.e.m.) percent reduction in Ca 2+ transient tail integral ([T 40 −T 10 ] × 100) for the experiments shown in g . * P <0.05 compared with control by analysis of variance and post hoc Student–Newman–Keuls test. Full size image In FDB fibres perfused with control Ringer’s solution, peak tetanic Ca 2+ transient amplitude decreased progressively from the first train, reaching ~50% by the 60th train ( Fig. 3a ). In the presence of 0.2 mM LaCl 3 plus 0.5 mM CdCl 2 (La/Cd), the amplitude of the first tetanic Ca 2+ transient was not significantly different from that observed in control, consistent with the independence of skeletal muscle EC coupling on Ca 2+ entry. However, the decrement in tetanic Ca 2+ transient magnitude was significantly greater by the 30th train, and even more so by the 60th train, in the presence of La/Cd ( Fig. 2a and Supplementary Fig. S2b ). As a result, a clear sustained phase of Ca 2+ transient amplitude was observed between T10 and T40 under control conditions (−4.3±2.8%, average±s.e.m.) that was reduced approximately sevenfold in the presence of La/Cd (−29.9±2.8%; Fig. 3b ). Similarly, the tail Ca 2+ transient integral, which reflects a balance between Ca 2+ influx and removal and increased (+10.2±9.6%, average±s.e.m.) between T40 and T10 in control (T40−T10), was reduced in the presence of La/Cd (−21.7±6.2%; Fig. 3c,d ). As La/Cd blocks multiple forms of Ca 2+ entry, effects of more targeted SOCE interventions were also determined. A similar accelerated reduction in peak Ca 2+ transient amplitude ( Fig. 3a,b ) and tail integral ( Fig. 3c,d ) during repetitive tetanic stimulation was observed following addition of SOCE channel inhibitors SK&F-96365 (30 μM) and BTP-2 (10 μM). Most importantly, a faster decay in peak Ca 2+ transient amplitude ( Fig. 3e,f ) and tail Ca 2+ transient integral ( Fig. 3g,h ) was also observed in FDB fibres following STIM1 knockdown (but not for control siRNA) and transient expression of Orai1E108Q mutant. The results in Fig. 3 indicate that SOCE has an important role in maintaining Ca 2+ transient amplitude during repetitive, high-frequency tetanic stimulation. Characterization of muscle-specific dnOrai1 transgenic mice SOCE is abolished in myotubes [12] and FDB fibres following transient expression of Orai1E108Q ( Fig. 2e,h ). Therefore, to investigate the role of Orai1-dependent Ca 2+ entry in adult skeletal muscle, we generated muscle-specific dnOrai1 (E108Q) transgenic mice ( Fig. 4a ; see Methods). Several transgenic lines exhibiting either low (line 102), medium (line 5) or high but variable (line 86) dnOrai1 expression were generated ( Fig. 4b ). Expression of the dnOrai1 protein assessed using an anti-haemagglutinin (HA) antibody was highly skeletal muscle specific, with no detectable expression in the heart, spleen, liver, lung or kidney ( Fig. 4c ). The dnOrai1 protein was partially glycosylated as the doublet band observed on western blot was consolidated to a single band following de-glycosylation with PNGaseF ( Fig. 4c ). Immunocytochemistry of FDB fibres from line-5 mice using an anti-HA antibody showed a double-rowed striated pattern that co-localized with STIM1 fluorescence ( Fig. 4d ), similar to that observed for endogenous Orai1 ( Fig. 1a ). Importantly, FDB fibres obtained from both line-86 ( Fig. 4e,f ) and line-5 ( Fig. 4f ) mice lacked SOCE as assessed by Mn 2+ quench. 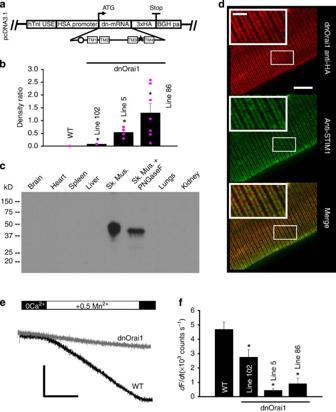Figure 4: Generation of muscle-specific dnOrai1 transgenic mice. (a) Schematic representation of the transgene vector used to create multiple lines of muscle-specific dnOrai1 mice. The dominant-negative E108Q point mutation and a C-terminal 3 × HA epitope were engineered into a mouse Orai1 cDNA and then cloned into a transgene vector containing a human troponin I upstream enhancer (hTnIUSE), a human skeletal muscle actin (HSA) promoter and a 3′ bovine growth hormone polyadenylation (BGHpa) tail. (b) Relative HA-tagged dnOrai1 protein expression in TA muscles from WT (n=3) and dnOrai1 transgenic lines 102 (n=3), 5 (n=4) and 86 (n=7) probed by an anti-HA antibody using western blot analysis. HA immunoreactivity was normalized to SERCA. Pink filled circles () indicate the relative expression of dnOrai1 in every individual mouse analysed. *P<0.05 by analysis of variance followed by Dunn’spost hoctest. Line-5 mice exhibit uniform moderate transgene expression, whereas line-86 mice exhibit high but more variable tansgene expression. (c) Western blot analysis with an anti-HA antibody showing skeletal muscle-specific expression of dnOrai1 protein in line-5 mice. (d) Imunonocytochemical labelling of dnOrai1 with anti-HA antibody (top), endogenous STIM1 (middle) and a merged image showing co-localization of the two proteins in double rows of striated fluorescence reflecting triad distribution (bottom). Scale bar, 10 μm. (e) Representative Mn2+quench traces in TG-treated FDB fibres obtained from WT and line-86 dnOrai1 mice. Scale bars, 100 s (horizontal), 4 × 105counts (vertical). (f) Average (±s.e.m.) maximum rate of Mn2+quench in TG-treated FDB fibres from WT (n=9), line-102 (n=13), line-5 (n=15) and line-86 (n=7) dnOrai1 mice. *P<0.05 compared with WT by Student’st-test. Figure 4: Generation of muscle-specific dnOrai1 transgenic mice. ( a ) Schematic representation of the transgene vector used to create multiple lines of muscle-specific dnOrai1 mice. The dominant-negative E108Q point mutation and a C-terminal 3 × HA epitope were engineered into a mouse Orai1 cDNA and then cloned into a transgene vector containing a human troponin I upstream enhancer (hTnIUSE), a human skeletal muscle actin (HSA) promoter and a 3′ bovine growth hormone polyadenylation (BGHpa) tail. ( b ) Relative HA-tagged dnOrai1 protein expression in TA muscles from WT ( n =3) and dnOrai1 transgenic lines 102 ( n =3), 5 ( n =4) and 86 ( n =7) probed by an anti-HA antibody using western blot analysis. HA immunoreactivity was normalized to SERCA. Pink filled circles ( ) indicate the relative expression of dnOrai1 in every individual mouse analysed. * P <0.05 by analysis of variance followed by Dunn’s post hoc test. Line-5 mice exhibit uniform moderate transgene expression, whereas line-86 mice exhibit high but more variable tansgene expression. ( c ) Western blot analysis with an anti-HA antibody showing skeletal muscle-specific expression of dnOrai1 protein in line-5 mice. ( d ) Imunonocytochemical labelling of dnOrai1 with anti-HA antibody (top), endogenous STIM1 (middle) and a merged image showing co-localization of the two proteins in double rows of striated fluorescence reflecting triad distribution (bottom). Scale bar, 10 μm. ( e ) Representative Mn 2+ quench traces in TG-treated FDB fibres obtained from WT and line-86 dnOrai1 mice. Scale bars, 100 s (horizontal), 4 × 10 5 counts (vertical). ( f ) Average (±s.e.m.) maximum rate of Mn 2+ quench in TG-treated FDB fibres from WT ( n =9), line-102 ( n =13), line-5 ( n =15) and line-86 ( n =7) dnOrai1 mice. * P <0.05 compared with WT by Student’s t -test. Full size image Unlike that observed following global or muscle-specific STIM1 ablation [11] , [13] , line-5 muscle-specific dnOrai1 transgenic mice were born at normal Mendelian ratios, thrived into adulthood and exhibited normal activity and fertility during the course of study up to 10 months of age. Similar to STIM1 knockout mice, line-5 dnOrai1 mice exhibited a significant reduction in whole-body mass at birth compared with wild-type (WT) littermates, which persisted throughout postnatal development and into adulthood ( Fig. 5a ). Muscle mass of tibialis anterior (TA), extensor digitorum longus (EDL) and soleus muscles were all significantly reduced (~20–30%) in line-5 dnOrai1 mice compared with WT littermates ( Fig. 5 b). Analysis of muscle cross-sectional area (CSA) by dystrophin immunolabelling revealed a significant reduction (~33%) in average fibre CSA in TA muscles of line-5 dnOrai1 mice ( Fig. 5c,d ). Nevertheless, haematoxylin and eosin (H&E) staining of TA muscle sections showed no evidence of muscle damage, degeneration, central nucleation or infiltration of inflammatory fibres from line-5 dnOrai1 mice ( Fig. 5c , bottom). In addition, myosin heavy chain analyses revealed no change in the proportion of type I, IIa, IIx or IIb fibres in TA, EDL, soleus and FDB muscles ( Fig. 5e,f ). Using electron microscopy, the ultrastructure, myofibril spacing and disposition of SR, transverse tubules, triads and the mitochondria in EDL and FDB fibres from line-5 dnOrai1 mice were indistinguishable from WT (see Fig. 6 for additional details). Only a few fibres from line-5 dnOrai1 mice (3/63) exhibited minor structural defects (limited regions of Z-line streaming or a few swollen mitochondria). 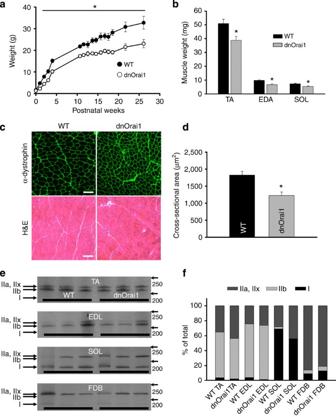Figure 5: Reduced weight and fibre CSA in dnOrai1 transgenic mice. (a) Postnatal growth curves (birth to 6 months) obtained from line-5 mice showing a significant reduction in total body weight of muscle-specific dnOrai1 transgenic mice compared with WT littermate controls (n=5 female mice with both WT and dnOrai1). *P<0.01 compared with WT by Student’st-test. (b) Average (±s.e.m.) muscle weight of TA, EDL and soleus in line-5 dnOrai1 transgenic mice (n=5 mice) compared with that of WT littermate controls (n=7 mice). *P<0.05 compared with corresponding WT control by Student’st-test. (c) Representative dystrophin immunostaining (top panel) and H&E images (bottom panel) of TA muscle cross-sections from WT and line-5 dnOrai1 mice. Scale bars, 100 μm. (d) Average (±s.e.m.) fibre CSA calculated from dystrophin-stained TA muscle (as shown inc) from WT (n=4) and line-5 dnOrai1 mice (n=3). *P<0.05 by Student’st-test. (e) Representative silver-stained polyacrylamide gel images of myosin heavy chain analysis from TA, EDL soleus and FDB of three different WT and line-5 dnOrai1 mice. Molecular weight markers are indicated to the right of each gel. (f) Stacked bar graph showing average fast IIa, IIx, IIb and slow type I fibre composition in WT and line-5 dnOrai1 transgenic mice (n=3–5 for both WT and dnOrai1). No significant difference in fibre-type composition was observed between WT and dnOrai1 mice. Figure 5: Reduced weight and fibre CSA in dnOrai1 transgenic mice. ( a ) Postnatal growth curves (birth to 6 months) obtained from line-5 mice showing a significant reduction in total body weight of muscle-specific dnOrai1 transgenic mice compared with WT littermate controls ( n =5 female mice with both WT and dnOrai1). * P <0.01 compared with WT by Student’s t -test. ( b ) Average (±s.e.m.) muscle weight of TA, EDL and soleus in line-5 dnOrai1 transgenic mice ( n =5 mice) compared with that of WT littermate controls ( n =7 mice). * P <0.05 compared with corresponding WT control by Student’s t -test. ( c ) Representative dystrophin immunostaining (top panel) and H&E images (bottom panel) of TA muscle cross-sections from WT and line-5 dnOrai1 mice. Scale bars, 100 μm. ( d ) Average (±s.e.m.) fibre CSA calculated from dystrophin-stained TA muscle (as shown in c ) from WT ( n =4) and line-5 dnOrai1 mice ( n =3). * P <0.05 by Student’s t -test. ( e ) Representative silver-stained polyacrylamide gel images of myosin heavy chain analysis from TA, EDL soleus and FDB of three different WT and line-5 dnOrai1 mice. Molecular weight markers are indicated to the right of each gel. ( f ) Stacked bar graph showing average fast IIa, IIx, IIb and slow type I fibre composition in WT and line-5 dnOrai1 transgenic mice ( n =3–5 for both WT and dnOrai1). No significant difference in fibre-type composition was observed between WT and dnOrai1 mice. 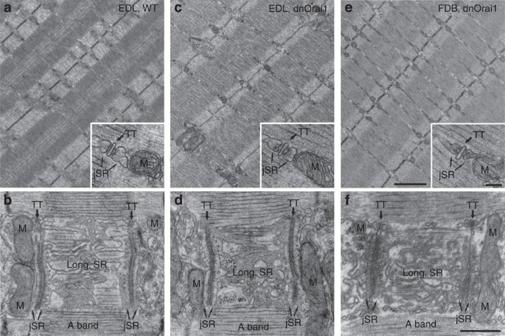Figure 6: Preserved skeletal muscle ultrastructure in EDL and FDB muscle of line-5 dnOrai1 mice. Representative electron microscopy micrographs from WT EDL (a,b), line-5 dnOrai1 EDL (c,d) and line-5 dnOrai1 FDB (e,f), with all samples exhibiting similar ultrastructure. Sarcomeres of adjacent myofibrils are similarly well aligned (a,c,e), with triads and the mitochondria closely associated (insets). Junctional SR (jSR) is closely associated with transverse tubules (TT) adjacent to the sarcomere I–A band transition, whereas longitudinal SR (long. SR) is placed at the A band (images are close to the surface of a myofibril;b,d,f). Mitochondria (M) are in close proximity of jSR/TT junctions (triads) on the side opposite to long. SR in fibres from both WT (b) and dnOrai1 (d,f) mice. Scale bars, 1 μm (a,c,e); 0.5 μm (b,d,f); 0.1 μm (insets). Full size image Figure 6: Preserved skeletal muscle ultrastructure in EDL and FDB muscle of line-5 dnOrai1 mice. Representative electron microscopy micrographs from WT EDL ( a , b ), line-5 dnOrai1 EDL ( c , d ) and line-5 dnOrai1 FDB ( e , f ), with all samples exhibiting similar ultrastructure. Sarcomeres of adjacent myofibrils are similarly well aligned ( a , c , e ), with triads and the mitochondria closely associated (insets). Junctional SR (jSR) is closely associated with transverse tubules (TT) adjacent to the sarcomere I–A band transition, whereas longitudinal SR (long. SR) is placed at the A band (images are close to the surface of a myofibril; b , d , f ). Mitochondria (M) are in close proximity of jSR/TT junctions (triads) on the side opposite to long. SR in fibres from both WT ( b ) and dnOrai1 ( d , f ) mice. Scale bars, 1 μm ( a , c , e ); 0.5 μm ( b , d , f ); 0.1 μm (insets). Full size image Western blot analysis using an Orai1-specific antibody showed no change in endogenous Orai1 expression in TA muscles of dnOrai1 mice ( Supplementary Fig. S3a ). Expression of STIM1 ( Supplementary Fig. S3b ) and other proteins involved in Ca 2+ homoeostasis (that is, sarco/endoplasmic Ca 2+ ATPase 1, RyR1, calsequestrin type 1 and dihydropyridine receptor α1-subunit; Supplementary Fig. S4 ) were also unaltered in TA muscles of dnOrai1 mice. Consistent with this, the magnitude and decay kinetics of electrically evoked twitch Ca 2+ release was not different in single FDB fibres from adult WT and dnOrai1 mice ( Supplementary Fig. S5a–c ). However, total Ca 2+ store content assessed using a rapid Ca 2+ store release cocktail [33] was significantly reduced ( P <0.01, Student’s t -test) in FDB fibres from dnOrai1 mice (fura-2FF Δratio was 0.36±0.03, average±s.e.m. n =11 and 0.17±0.05, n =6 for WT and dnOrai1, respectively; Supplementary Fig. S5d,e ). dnOrai1 mice exhibit increased susceptibility to fatigue As muscle-specific dnOrai1 mice thrive into adulthood and lack SOCE in skeletal muscle ( Fig. 4e,f ), these mice provide a unique opportunity to determine the physiological role of Orai1-dependent SOCE in adult muscle. As an initial test of the functional impact of loss of SOCE in muscle, we compared ex vivo muscle contractility of EDL muscles isolated from 4–6-month old WT and line-5 dnOrai1 mice. The magnitude and kinetics of EDL twitch contraction were not different between WT and dnOrai1 ( Fig. 7a , left traces), consistent with the normal fibre-type distribution, ultrastructure and EC coupling in muscles from dnOrai1 mice. However, a modest reduction in peak muscle-specific force was observed in EDL muscles from dnOrai1 mice at stimulation frequencies ≥100 Hz ( Fig. 7a,b ). EDL muscles from dnOrai1 mice also exhibited a reduced ability to maintain contractile force at high frequencies during each 500 ms stimulation ( Fig. 7a , grey traces and Fig. 7c), consistent with an increase in EDL fatigability during intense stimulation. Moreover, the magnitude of force decay during a prolonged tetanus (150 Hz, 2 s) was increased in EDL muscles from dnOrai1 mice ( Fig. 7d,e ). 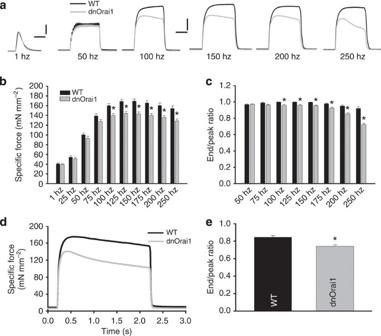Figure 7: Altered maximum tetanic-specific force and contractile decay in EDL muscles of dnOrai1 mice. (a) Representative superimposed contraction traces elicited at different stimulation frequencies (1, 50, 100, 150, 200 and 250 Hz) in EDL muscles from WT (black) and line-5 dnOrai1 (grey) mice. (b) Frequency dependence of average (±s.e.m.) specific force (mN mm−2) in EDL muscles from WT (black,n=14) and line-5 dnOrai1 mice (grey,n=14). *P<0.01 compared with corresponding control by Student’st-test. (c) Frequency dependence of average (±s.e.m.) contractile decay (end/peak ratio) for EDL muscles from WT (black bars,n=14) and line-5 dnOrai1 (grey bars,n=14). *P<0.01 compared with corresponding control by Student’st-test. (d,e) Representative contractile traces (d) and average contractile decay (end/peak ratio;e) during a single 2 s, 150 Hz stimulation train in EDL muscles from WT (black,n=10) and line-5 dnOrai1 mice (grey,n=11). *P<0.01 compared with WT by Student’st-test. Scale bars, 50 ms (left, for twitch only, horizontal); 20 mN mm−2(vertical); 200 ms (right, for tetani, horizontal); 50 mN mm−2(vertical). Figure 7: Altered maximum tetanic-specific force and contractile decay in EDL muscles of dnOrai1 mice. ( a ) Representative superimposed contraction traces elicited at different stimulation frequencies (1, 50, 100, 150, 200 and 250 Hz) in EDL muscles from WT (black) and line-5 dnOrai1 (grey) mice. ( b ) Frequency dependence of average (±s.e.m.) specific force (mN mm −2 ) in EDL muscles from WT (black, n =14) and line-5 dnOrai1 mice (grey, n =14). * P <0.01 compared with corresponding control by Student’s t -test. ( c ) Frequency dependence of average (±s.e.m.) contractile decay (end/peak ratio) for EDL muscles from WT (black bars, n =14) and line-5 dnOrai1 (grey bars, n =14). * P <0.01 compared with corresponding control by Student’s t -test. ( d , e ) Representative contractile traces ( d ) and average contractile decay (end/peak ratio; e ) during a single 2 s, 150 Hz stimulation train in EDL muscles from WT (black, n =10) and line-5 dnOrai1 mice (grey, n =11). * P <0.01 compared with WT by Student’s t -test. Scale bars, 50 ms (left, for twitch only, horizontal); 20 mN mm −2 (vertical); 200 ms (right, for tetani, horizontal); 50 mN mm −2 (vertical). Full size image We next compared the ability of muscles from dnOrai1 mice to produce sustained Ca 2+ release and force production during repetitive high-frequency tetanic stimulation ( Fig. 8a–d ). Single FDB fibres from WT and dnOrai1 mice were subjected to the same repetitive tetanic stimulation train used for the experiments shown in Fig. 3 (50 Hz, 500 ms, every 2.5 s, 60 times). Consistent with results obtained with SOCE channel inhibitors, STIM1 KD, and Orai1E108Q expression, peak tetanic Ca 2+ transient decline was accelerated in FDB fibres from dnOrai1 mice ( Fig. 8a ). Peak Ca 2+ transient amplitude decreased 47.0±7.3% (average±s.e.m.) from T5 to T40 in fibres from dnOrai1 mice, in contrast to only 15.6±9.6% for fibres from WT mice ( Fig. 8b ). A similar accelerated decline in force production repetitive tetanic stimulation was also observed in EDL muscles from dnOrai1 mice ( Fig. 8c ) where tetanic force during the first five tetani decreased 14.6±2.7% (average±s.e.m.) for dnOrai1 compared with only 7.4±1.6% for WT ( Fig. 8d ). A similar decrease in peak-specific force and increased fatigability during repetitive stimulation were observed in EDL muscles from dnOrai1 line-86 mice ( Supplementary Fig. S6 ) Altogether, these results are consistent with a significant contribution of SOCE to sustained Ca 2+ release and force production during repetitive, high-frequency stimulation. 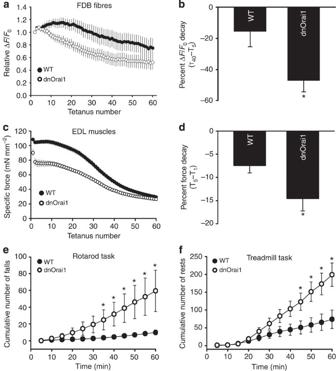Figure 8: dnOrai mice exhibit increased susceptibility to fatigue. (a) Average (±s.e.m.) peak Ca2+transient amplitude during 60 consecutive tetanic stimuli (500 ms at 50 Hz every 2.5 s) in FDB fibres obtained from either WT (filled circles,n=11) or line-86 dnOrai1 transgenic mice (open circles,n=15). (b) Average (±s.e.m.) percent reduction in peak Ca2+transient amplitude from tetanus 5 to tetanus 40 ([T40−T5] × 100) for the experiments shown ina. *P<0.05 by Student’st-test. (c) Average (±s.e.m.) peak-specific force during 60 consecutive tetanic stimuli (500 ms, at 50 Hz, every 2.5 s) in EDL muscles from WT (filled circles,n=8 muscles from four mice) or line-5 dnOrai1 mice (open circles,n=8 muscles from five mice). (d) Average (±s.e.m.) percent force decay during the first five successive tetani (100 × [T5−T1]/T1) for the experiments shown inc. *P<0.05 by Student’st-test. (e) Average (±s.e.m.) cumulative number of falls during 1 h Rotarod endurance task in 4-month-old adult WT (n=11) and line-5 dnOrai1 (n=9) mice (see Methods). *P<0.05 by Student’st-test. (f) Average (±s.e.m.) cumulative number of rests (that is, all four paws off the treadmill) observed during 1 km treadmill run in 4-month-old adult WT (n=6) and line-5 dnOrai1 (n=5) mice (see Methods). *P<0.05 by Student’st-test. The phenotypes (absence of SOCE, reduced body and muscle weight, increased fatigue, reduced treadmill running) of line-5 mice on the mixed background (B6SJL hybrid) was the same as that observed for line-5 mice following backcross onto a congenic C57Bl6 background. Figure 8: dnOrai mice exhibit increased susceptibility to fatigue. ( a ) Average (±s.e.m.) peak Ca 2+ transient amplitude during 60 consecutive tetanic stimuli (500 ms at 50 Hz every 2.5 s) in FDB fibres obtained from either WT (filled circles, n =11) or line-86 dnOrai1 transgenic mice (open circles, n =15). ( b ) Average (±s.e.m.) percent reduction in peak Ca 2+ transient amplitude from tetanus 5 to tetanus 40 ([T 40 −T 5 ] × 100) for the experiments shown in a . * P <0.05 by Student’s t -test. ( c ) Average (±s.e.m.) peak-specific force during 60 consecutive tetanic stimuli (500 ms, at 50 Hz, every 2.5 s) in EDL muscles from WT (filled circles, n =8 muscles from four mice) or line-5 dnOrai1 mice (open circles, n =8 muscles from five mice). ( d ) Average (±s.e.m.) percent force decay during the first five successive tetani (100 × [T 5 −T 1 ]/T 1 ) for the experiments shown in c . * P <0.05 by Student’s t -test. ( e ) Average (±s.e.m.) cumulative number of falls during 1 h Rotarod endurance task in 4-month-old adult WT ( n =11) and line-5 dnOrai1 ( n =9) mice (see Methods). * P <0.05 by Student’s t -test. ( f ) Average (±s.e.m.) cumulative number of rests (that is, all four paws off the treadmill) observed during 1 km treadmill run in 4-month-old adult WT ( n =6) and line-5 dnOrai1 ( n =5) mice (see Methods). * P <0.05 by Student’s t -test. The phenotypes (absence of SOCE, reduced body and muscle weight, increased fatigue, reduced treadmill running) of line-5 mice on the mixed background (B6SJL hybrid) was the same as that observed for line-5 mice following backcross onto a congenic C57Bl6 background. Full size image Finally, dnOrai1 mice were used to assess the consequences of loss of SOCE function on muscle performance at the whole-animal level. Age- (4–5-month-old male) and sex-matched WT and line-5 dnOrai1 mice were evaluated using a prolonged Rotarod protocol designed to assess endurance. In this test, mice were placed on a motor driven Rotarod wheel and forced to walk on the rotating wheel for 2 h while the speed was increased modestly at regular intervals (see Methods). WT mice remained on the wheel with only a few falls during the first hour, with progressively more falls during the second hour. On the other hand, although initially performing equally well at the task, dnOrai1 mice exhibited a significant increase in the number of cumulative falls compared with WT mice at all times 30 min after initiation of the task ( Fig. 8e and Supplementary Movie 1 ). Because of exhaustion, several dnOrai1 mice were unable to complete the entire 2 h protocol. Thus, only the cumulative number of falls during the first 60 min of the task is shown in Fig. 8e . As a second measure of fatigue, a separate group of WT and line-5 dnOrai1 mice were subjected to three consecutive days of acute treadmill running (see Methods). All WT and dnOrai1 mice completed the entire 1 km run on each of three consecutive days. However, WT mice completed the task with limited rests and encouragement. On the other hand, after approximately the first 40 min of running, dnOrai1 mice exhibited a significant increase in the number of rests and required more encouragement to re-engage the treadmill and continue running ( Fig. 8f and Supplementary Movie 2 ). Altogether, results from the Rotarod exhaustion and treadmill-running tasks indicate that adult dnOrai1 mice exhibit a significantly increased susceptibility to muscle fatigue. This study characterized the structural basis and physiological role of SOCE in adult skeletal muscle. Immunocytochemical results provide direct evidence for co-localization of endogenous Orai1 and STIM1 in the triad junction and Mn 2+ quench studies found that STIM1–Orai1 coupling is required for SOCE in adult skeletal muscle. This close disposition of STIM1 and Orai1 in existing SR-T-tubule triad junctions enables rapid SOCE activation as STIM1 and SR redistribution following store depletion is not required. However, results of BiFC experiments indicate that preformed STIM1–Orai1 complexes are not present in resting muscle fibres with fully replete SR Ca 2+ stores and that store depletion is required to drive the formation of junctional Orai1–STIM1 complexes. FRET-based studies will be required to further resolve the time course of junctional STIM1–Orai1 complex formation during SR Ca 2+ store depletion. The survival of muscle-specific dnOrai1 mice allowed us to assess the physiological role of Orai1-dependent SOCE in adult skeletal muscle. Although line-5 dnOrai1 mice lack SOCE, these mice thrive into adulthood and exhibit normal muscle histology and fibre-type distribution. Thus, Orai1-dependent SOCE is clearly not required for survival. However, as muscle mass and CSA are reduced in line-5 dnOrai1 mice, SOCE is required for normal muscle growth. Although high expressing line-86 mice are fertile, live well into adulthood and exhibit a similar reduction in muscle mass and CSA, some of these mice exhibit histopathological signs of myopathy including increased cell infiltration, central nucleation and the development of kyphosis at advanced ages. The myopathic phenotypes observed in line-86 mice is unlikely due to loss of Orai1-dependent SOCE, as they are not observed in line-5 mice that also lack SOCE. The reasons for the variable myopathic alterations observed in line-86 dnOrai1 mice is unclear but may involve off-target effects (for example, inhibition of TrpC channels) [34] of the high level of dnOrai1 expression observed in some of these mice ( Fig. 4b ). The role of SOCE in refilling SR Ca 2+ stores in skeletal muscle is controversial. On the one hand, SR Ca 2+ content was reported to be increased in FDB fibres from mdx mice [35] where Orai1 [35] , [36] and STIM1 (ref. 36 ) protein levels are upregulated and SOCE is enhanced, whereas SR Ca 2+ store content is reduced in muscle-specific STIM1 knockout mice that lack SOCE [11] . However, as other critical Ca 2+ -handling proteins (for example, SERCA, TrpC3/6 and NCX3) are also altered in these models [11] , [35] , the specific role of STIM1–Orai1 coupling in store refilling remains unclear. In addition, Launikonis et al . [25] reported that in spite of changes in STIM1 and Orai1 expression in mdx muscle, SR Ca 2+ content was unaltered in mechanically skinned EDL muscle fibres [36] , and thus concluded that SOCE has little or no role in refilling SR Ca 2+ stores in skeletal muscle [25] , [36] , [37] . However, as SR reloading in mechanically skinned fibres may be different from that of intact fibres, the relevance of these results to Ca 2+ store content in intact fibres under more physiological conditions is unclear. Our finding that resting Ca 2+ store content was significantly reduced in intact single FDB fibres from dnOrai1 mice is consistent with Orai1-dependent Ca 2+ entry having a role in maintaining and refilling SR Ca 2+ stores as it does in non-excitable cells. In addition, as no alterations in other major Ca 2+ -handling proteins were found in the muscle from dnOrai1 mice ( Supplementary Fig. S4 ), our findings provide the strongest evidence to date that Orai1-dependent SOCE contributes to store refilling in the skeletal muscle. The reduction in total Ca 2+ store content likely contributes to the reduced peak tetanic-specific force and accelerated fatigue with repetitive high-frequency stimulation. During repetitive tetanic stimulation of FDB fibres from WT mice, peak Ca 2+ transient magnitude is maintained and Ca 2+ transient tail integral is increased, both of which are reduced by SOCE inhibitors, STIM1 KD, and dnOrai1 expression. These findings indicate that repetitive tetanic stimulation promotes store depletion and activation of STIM1/Orai1-dependent SOCE needed to replenish SR Ca 2+ stores and maintain Ca 2+ release during subsequent tetani. Thus, SOCE has an important role in sustaining Ca 2+ release and contractile force during repetitive tetanic stimulation, consistent with that reported previously when SOCE activity is reduced either pharmacologically [19] or in aging [38] . Our findings that adult dnOrai1 mice exhibit a marked increased susceptibility to exhaustion during prolonged Rotarod and treadmill exercise provide the strongest evidence to date that Orai1-dependent SOCE has a key role in limiting muscle fatigue during strenuous exercise. Muscle-specific dnOrai1 transgenic mice also provide insight into the role of Orai1-dependent SOCE in skeletal muscle development, specification, growth and survival. As reported for muscle-specific STIM1 knockout mice [11] , dnOrai1 mice exhibit similar reductions in body weight, muscle mass and fibre CSA. Taken together, these findings demonstrate that STIM1–Orai1 signalling promotes muscle growth in both young and adult mice, presumably through the activation of Ca 2+ -dependent downstream signalling cascades [11] . However, STIM1 knockout mice also exhibit hypotonia, increased central nucleation, swollen mitochondria and neonatal lethality [11] , [13] , none of which are observed in line-5 dnOrai1 mice. These additional phenotypes observed in STIM1 knockout mice, but not in line-5 dnOrai1 mice, probably reflect altered activity of one or more non-Orai1 STIM1 targets including TrpC/ARC/Ca V channels, SERCA/PMCA/NCX pumps/exchangers, adaptor proteins, ER chaperones, second messenger enzymes or ER stress/remodelling proteins [23] . In summary, we provide a comprehensive characterization of Orai1-dependent SOCE in adult skeletal muscle. SOCE in adult muscle depends on junctional STIM1–Orai1 coupling, which is important for both normal muscle growth and susceptibility to fatigue. Altered SOCE activity has been proposed to contribute to muscle dysfunction in various pathophysiological states of muscle including sarcopenia [38] , muscular dystrophy [36] and malignant hyperthermia [39] . Muscle-specific dnOrai1 mice will provide a powerful model to assess the relative importance of Orai1-dependent SOCE in normal muscle physiology and how SOCE dysfunction contributes to these and other muscle pathologies. In vivo electroporation of FDB muscles All experiments were approved by the University of Rochester Committee on Animal Recourses. Four to six-month-old male and female WT C57Bl6 mice were anaesthetized by intraperitoneal injection of 100 mg kg −1 ketamine, 10 mg kg −1 xylazine and 3 mg kg −1 acepromazine. Hindlimb footpads of anaesthetized mice were then injected with bovine hyaluronidase (10 μl, 0.4 U μl −1 ). One hour later, hindlimb footpads were subcutaneously injected with either cherry-tagged Orai1 cDNA construct (20 μg in 71 mM NaCl), STIM1-specific siRNAs (Dharmacon siGENOME SMARTpool, 20 pmol in 71 mM NaCl) or negative control siRNA (Dharmacon, 20 pmol in 71 mM NaCl, see Supplementary Table S1 for sequence) using a 30-gauge needle. The footpad was then electroporated with 10 stimulations of 100 V cm −1 , 20-ms duration delivered at 1 Hz using subcutaneous gold-plated electrodes placed perpendicular to the long axis of the muscle, close to the proximal and distal tendons [40] . FDB muscles and fibres were used for experiments either 5–8 days after cDNA injection or boosted with a second round of siRNA electroporation on day 5–7 and then used for experiments 10–12 days after the initial electroporation. Isolation of FDB muscle fibres FDB muscle fibres were dissociated from FDB muscles from 4–6-month-old male and female mice by enzymatic digestion in 0.1% collagenase A, 45 min at 37 °C in Ringer’s solution [40] . Bimolecular fluorescence complementation BiFC is based on the association of two non-fluorescent fragments of YFP that fuse together to form a functional fluorophore when the fragments were located in close proximity (within 10 nm) to each other [28] , [29] , [30] . Thus, a putative interaction between two proteins can be examined by attaching complementary YFP fragments to the two proteins with YFP fluorescence used as a read-out of the interaction. For these experiments, YFP was split into two fragments at amino acid 158. The amino-terminal fragment of YFP (1–158) was fused to the carboxy terminus of cherry-tagged STIM1 and the C-terminal YFP fragment (159–238) was fused to the C terminus of cherry-tagged Orai1 ( Supplementary Fig. 2A ). Cherry-STIM1-YFP1-158 and cherry-Orai1-YFP159-238 cDNAs were electroporated into mouse footpads at a 1:1 ratio. YFP fluorescence was monitored in cherry-expressing FDB fibres before and after store depletion. YFP and cherry were excited sequentially by 488 or 543 nm lasers, respectively, and fluorescence emission detected at 515/30 or 605/75 nm, respectively, with a Nikon Eclipse C1 Plus Confocal microscope (Nikon Instruments, Melville, NY, USA) using either SuperFluor × 40 (1.3 numerical aperture (NA)) or × 60 (1.4 NA) oil-immersion objectives. Images were analysed using AutoQuant software. Mn 2+ quench measurements Acutely isolated single FDB fibres were loaded with 5 μM fura-2 AM for 1 h at 37 °C in a Ca 2+ -free rodent Ringer’s solution containing (in mM): 145 NaCl, 5 KCl, 1 MgCl 2 , 10 HEPES, 0.2 EGTA, pH 7.4. During fura-2 loading, unless otherwise stated, all fibres were simultaneously treated with a SERCA pump inhibitor cocktail consisting of 1 μM TG, 15 μM cyclopiazonic acid (CPA) and 30 μM N -benzyl- p -toluene sulphonamide, a skeletal muscle myosin inhibitor used to inhibit movement during electrical stimulation, to deplete SR Ca 2+ stores, prevent Ca 2+ reuptake and activate SOCE. Store-depleted fibres were then plated on glass-bottom dishes, bathed in Ca 2+ -free Ringer’s and excited at 362 nm (isosbestic point of fura-2), while emission was detected at 510 nm using a DeltaRam illumination system (Photon Technology, Birmingham, NJ). After obtaining an initial rate of fura-2 quench from ( R baseline ), FDB fibres were then exposed to 0.5 mM MnCl 2 to access the rate of Mn 2+ entry. The maximum rate of fura-2 quench in the presence of Mn 2+ ( R max ) was then obtained from the peak differential of the fura-2 emission trace during Mn 2+ application. The rate of SOCE was calculated as R SOCE = R max − R baseline and expressed as d F/ d t in counts s −1 (ref. 12 ). High-frequency tetanic stimulation of FDB fibres Myoplasmic Ca 2+ transient in FDB fibres during high-frequency tetanic stimulation were monitored using mag-fluo-4 (ref. 41 ) throughout the entire repetitive tetanic stimulation train (60 successive 500 ms, 50 Hz tetani every 2.5 s; Supplementary Fig. S2a , top). FDB fibres were perfused with Ringer’s solution in the presence or absence of Ca 2+ influx blockers. Peak Ca 2+ transient amplitude was measured at the end of each tetani and expressed as ( F max − F 0 )/ F 0 ( Supplementary Fig. S2a ). The integral of the Ca 2+ transient decay following each tetanus was also calculated ( Supplementary Fig. S2a ). Average data were expressed as relative peak amplitudes and relative tail integrals to control for variability between cells. Orai1 cloning and generation of dnOrai1 mice Total RNA was extracted from mouse spleen using TRIZOL reagent according to the manufacturer’s instructions. Before reverse transcription, RNA was treated with DNAase I for 15 min at room temperature. RNA was then reverse transcribed using Superscript III reverse transcriptase and oligo dTs. Murine WT Orai1 DNA was cloned using PCR and sequence-specific primers. A single amino-acid dominant-negative mutation in murine Orai1 (E108Q) was introduced using standard two-step site-directed mutagenesis. Three consecutive HA epitope (3xHA) sequences were similarly inserted in-frame at the extreme Orai1 C terminus. The dnOrai1-3xHA construct was then cloned into a skeletal muscle-specific transgene vector containing a human troponin I enhancer, HSA (human skeletal muscle actin) promoter and a BGH (bovine growth hormone) polyadenylation signal (pcDNA3.1(+)-hTnI-HSA-BGHpA (gift from Dr Jeffery D. Molkentin) [42] . The vector was linearized and injected into pronuclei of fertilized mouse oocytes by the University of Rochester Medical Center transgenic core facility. Founder lines exhibiting different levels of transgene incorporation were generated in a mixed background (B6SJL hybrid). Line-5 mice, exhibiting medium level of muscle-specific dnOrai1 protein expression ( Fig. 3 ), were then backcrossed into C57Bl6 background. Genotyping was performed by PCR using the following primers: forward: 5′-CAAGTCCAGCTCGACACAGA-3′ reverse: 5′-CTGCATAGTCCGGGACGTCATAGG-3′. Immunocytochemistry Freshly isolated FDB fibres were fixed with 4% paraformaldehyde and labelled/co-labelled using different primary antibodies (see Supplementary Table S2 for details) followed by appropriate Rhodamine/Alexa Fluor 488-conjugated secondary antibodies. Rhodamine and Alexa 488 were sequentially excited using 543 and 488 nm lasers, and detected at 605/75 and 515/30 nm, respectively, using a Nikon D-Eclipse C1 confocal microscope equipped with a × 40, NA 1.3 oil-immersion objective. Images were averaged ( n =4) and deconvolved (two-dimensional blind) for presentation. Immunohistochemistry and H&E staining of TA muscle Snap frozen TA muscles from WT and dnOrai1 mice were cut into 10 μm thick sections and probed using a mouse monoclonal anti-dystrophin antibody (MANDRA1, Abcam, 1:500). Sections were visualized using Alexa Fluor 488 anti-mouse antibody and imaged as described above (in Immunocytochemistry). Fibre CSA was calculated using ImageJ software. Similar sections were alternatively stained using H&E to assess muscle ultrastructure, specifically the presence of centrally nucleated fibres and fibrosis. Electron microscopy After killing, EDL and FDB muscles were fixed in situ at room temperature and maintained in fixative (3.5% glutaraldehyde in 0.1 M NaCaCo buffer, pH 7.2) until use. Small portions of muscle were post-fixed, embedded, stained en-block and sectioned [43] . Ultrathin sections (~50 nm), after staining in 4% uranyl acetate and lead citrate, were examined with a Morgagni Series 268D electron microscope (FEI Company, Brno, Czech Republic), equipped with Megaview III digital camera. Western blot analysis TA muscles were excised and homogenized in ice-cold RIPA buffer and centrifuged at 4 °C, 16,000 g for 15 min and supernatants were collected for analysis. Prepared sample were solubilized in standard Laemmli sample buffer before electrophoresis. Proteins were separated by SDS–polyacrylamide gel electrophoresis, transferred to nitrocellulose membrane and immunostained with different primary antibodies followed by appropriate horseradish peroxidase-conjugated secondary antibodies (see Supplementary Table S2 ). Blots were visualized by enhanced chemiluminescence. Protein band densities were quantified using ImageJ software, using either GAPDH or α-actinin as loading controls. Full-length images of immunoblots are shown in Supplementary Fig. S7 . Measurements of total SR Ca 2+ FDB fibres were loaded with 4 μM fura-2FF AM at room temperature for 30 min followed by a 30-min washout in dye-free Ringer’s solution. Total SR Ca 2+ content was determined by fura-2-FF fluorescence after local application of a Ca 2+ release cocktail (ICE-10 μM ionomycin, 30 μM cyclopiazonic acid and 100 μM EGTA/0 Ca 2+ ) [33] . Myosin heavy chain analysis TA, EDL, soleus and FDB muscles from 4–6-month-old male and female WT and dnOrai1 mice were homogenized on ice in a buffer containing (in mM) 20 imidazole (pH 7.2), 150 KCl and 0.2 EDTA with protease inhibitors. Tissue homogenates were centrifuged at 4 °C, 16,000 g for 15 min. Pellets were resuspended in a buffer containing (in mM) 50 Tris–HCl (pH 7.4), 150 NaCl with protease inhibitors, snap frozen and stored at 80 °C until use. Before analysis, prepared samples were diluted 1:1 in a sample buffer containing 0.16 M Tris–HCl (pH 6.8), 40% glycerol, 4% SDS, 0.1 M dithiothreitol and 0.02% bromophenol blue, and solubilized at 95 °C for 5 min. Myosin heavy chain isoforms were separated using SDS–polyacrylamide gel electrophoresis as described previously [44] , [45] with modifications. Electrophoresis were carried out using a Bio-Rad Mini Protean system, with resolving gels containing 8% acrylamide/bis (99:1), 35% glycerol, 0.4% SDS, 0.2 M Tris–HCl (pH 8.8), 0.1 M glycine, 0.1% ammonium persulfate, 0.05% N,N,N',N'-tetramethylethylenediamine and stacking gels containing 30% glycerol, 4% acrylamide/bis (49:1), 0.4% SDS, 70 mM Tris–HCl (pH 6.7), 4 mM EDTA, 0.1% ammonium persulfate and 0.05% N,N,N',N'-tetramethylethylenediamine. Protein (1.5 μg) was loaded in each lane. Gels were electrophoresed at 140 V for 16–18 h at 4 °C in running buffers containing: outer chamber, 0.05 M Tris, 0.075 M glycine 0.05% SDS; inner chamber: eight times the concentration of outer chamber supplemented with 0.12% β-mercaptoethanol. After electrophoresis, protein bands were visualized by silver staining, photographed, and relative composition of myosin heave chain isoforms were determined using ImageJ program. In vitro muscle contraction assay Muscle strength and fatigability were analysed in EDL muscles using an ASI muscle contraction system (Aurora Scientific), equipped with a 300C-LR dual mode force transducer and a 701C stimulator. Mice were anaesthetized by intraperitoneal injection of 100 mg kg −1 ketamine, 10 mg kg −1 xylazine and 2 mg kg −1 acepromazine. EDL muscles were exposed after removing TA muscles. The proximal and distal tendons of EDL muscle were then tied using 4-0 surgical suture, and EDL muscles were carefully excised and mounted between two platinum electrode plates while continuously perfused with oxygenated Ringer’s solution in the experimental chamber [46] . Muscle optimal length ( L o ) was determined using a series of 1 Hz stimulation and set at the length that generates the maximal force. Stimulus output was set at 120% of the voltage that elicits maximal force. Muscles were first equilibrated using three 500 ms, 150 Hz tetani at 1 min intervals and then subjected to a force frequency, a single sustained high-frequency tetanus (150 Hz, 2 s) and/or a repetitive tetanic fatiguing (60 successive 50 Hz, 500 ms tetani) protocol. Muscle force was recorded using a Dynamic Muscle Control software and analysed using Clampfit 10.0 software. Muscle CSA and specific force were calculated as described previously [46] . In vivo fatigue assays Rotarod and treadmill running were used to assess the fatigability of 4–6-month-old male and female WT and dnOrai1 mice during rigorous exercise. For rotarod endurance task, mice were first acclimated to rotarod running for 1 h on a Rotamex-5 (Columbus Instruments) at 15 r.p.m. for two consecutive days. On the following day, mice were placed on the rotarod at an initial speed of 15 r.p.m. for 15 min. The speed was then increased by 1 r.p.m. every 5 min for the following 30 min and then by 1 r.p.m. every 15 min for the rest of the 2-h task. In the event of a fall, the fall was noted and the mouse was returned to the rotarod. The number of cumulative falls over time during the task was recorded for each mouse. For treadmill (Columbus Instruments) experiments, mice were pre-trained for treadmill running 3 days before experiments, for 5 min each day at a speed of 5 m min −1 at a 15° inclination. An acute exhaustion protocol was used for the treadmill task. After a 5-min warm up at 5 m min −1 at a 15° inclination, treadmill speed was increased 1 m min −1 every minute up to 20 m min −1 and remained at the maximum speed for an additional 40 min. The entire task was 1 km in distance and 1 h in duration. Continued running was encouraged by delivering brief (<1 s) spirits of air on the mouse’s backside using a Whoosh Duster. The number of rests was recorded for each mouse. Finally, the number of cumulative falls (Rotarod) or cumulative rests (treadmill, binned every 5 min) across multiple animals for each genotype were then averaged and plotted against the duration of task. Data analysis Results are expressed as mean±s.e.m. with statistical significance determined using Student’s t -test for simple comparison and one-way analysis of variance followed by post hoc Student–Newman–Keuls test for multiple comparisons. P <0.05 were considered as statistically significant. How to cite this article: Wei-LaPierre, L. et al . Orai1-dependent calcium entry promotes skeletal muscle growth and limits fatigue. Nat. Commun. 4:2805 doi: 10.1038/ncomms3805 (2013).